Characterizing coral skeleton mineralogy with Raman spectroscopy 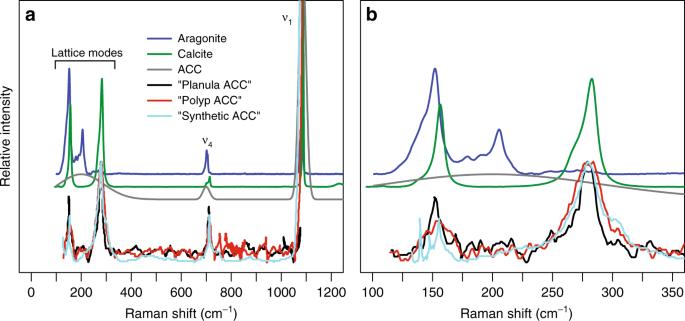Fig. 1 Reference Raman spectra of calcium carbonates: aragonite (blue), calcite (green), and ACC (gray).ashows the broad spectrum from 0 to 1300 cm−1that includes both lattice and internal modes, andbshows the narrower 100–400 cm−1lattice-mode region. Internal modes ν1and ν4are labelled, and the region of lattice modes for aragonite and calcite is indicated. The “Planula ACC” (black), “Polyp ACC” (red), and “Synthetic ACC” (cyan) lines show the data from Akiva et al.1interpreted as spectra of ACC. These three spectra all have distinct lattice mode peaks, clearly demonstrating they are not ACC, but rather a crystalline calcium carbonate consistent with calcite Reference aragonite and calcite spectra were acquired from the RRUFF online database (ID R080142 and R150075 , respectively) and plotted in Fig. 1 . An ACC spectrum (gray line in Fig. 1 ) was illustrated based on descriptions in the literature [7] , [13] , [14] of wide internal modes (e.g. ν 1 full width at half maximum intensity >20 cm −1 ) [7] , and an absence of distinct lattice mode peaks but with a broad background at <400 cm −1 due to some ordering of carbonate [13] . The corresponding authors of Akiva et al. [1] did not respond to requests for the raw Raman data, so their “ACC” spectra were extracted with the software Datathief ( http://www.datathief.org ). This was conducted on their Fig. 4 and their Supplementary Fig. 3 separately, and plotted here in Fig. 1a and Fig. 1b , respectively. In Fig. 1a , the Akiva et al. [1] data are only plotted below approximately 1080 cm −1 because it was not possible to extract the full ν 1 peak from their Fig. 4 since the spectra were overlapping.